Efficient palladium-catalyzed electrocarboxylation enables late-stage carbon isotope labelling 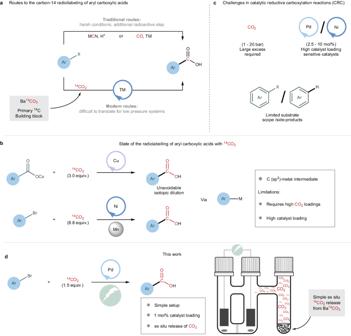Fig. 1: Radioactive labelling of aryl carboxylic acids. aComparison of using CO2, CO or MCN as carbon-14 sources for the radiolabelling of aryl carboxylic acids.bTop Modern dynamic CIE method limited to low-carbon isotope incorporations12. Bottom Modern strategy for radioactive CRC, limited to only one example and requiring high CO2loadings29.cChallenges in catalytic reductive carboxylation reactions (CRC).dProposed method for the late-stage palladium-catalysed electrocarboxylation of aryl electrophiles (this work). Carbon isotope labelling of bioactive molecules is essential for accessing the pharmacokinetic and pharmacodynamic properties of new drug entities. Aryl carboxylic acids represent an important class of structural motifs ubiquitous in pharmaceutically active molecules and are ideal targets for the installation of a radioactive tag employing isotopically labelled CO 2 . However, direct isotope incorporation via the reported catalytic reductive carboxylation (CRC) of aryl electrophiles relies on excess CO 2 , which is incompatible with carbon-14 isotope incorporation. Furthermore, the application of some CRC reactions for late-stage carboxylation is limited because of the low tolerance of molecular complexity by the catalysts. Herein, we report the development of a practical and affordable Pd-catalysed electrocarboxylation setup. This approach enables the use of near-stoichiometric 14 CO 2 generated from the primary carbon-14 source Ba 14 CO 3 , facilitating late-stage and single-step carbon-14 labelling of pharmaceuticals and representative precursors. The proposed isotope-labelling protocol holds significant promise for immediate impact on drug development programmes. The introduction of carbon isotopes ( 13 C and 14 C) into strategic positions of pharmaceutically active molecules is a crucial step for performing metabolic and pharmacokinetic studies (DMPK), the results of which ultimately determine their fate as potential drug candidates [1] , [2] . Similarly, in the search for new agrochemicals, their corresponding carbon isotopologues allow studies regarding metabolic profiling and the establishment of any possible human, soil, and groundwater contamination [3] , [4] , [5] . As such, it is imperative that efficient and accessible synthetic labelling technologies are at hand to facilitate late-stage installations of the isotope label into scaffolds of prospective drug entities. This provides rapid access to these essential isotopologues and avoids multiple manipulations of radioactive materials and waste for radiolabelling. Aryl carboxylic acids and their derivatives represent an example of a highly abundant structural motif in numerous bioactive structures [6] . Classical approaches for accessing their isotopically labelled variants include the carboxylation of preformed but reactive organometallic reagents or nitrile substitutions followed by hydrolysis (Fig. 1a ). Nevertheless, the harsh reaction conditions associated with such processes are characterised by poor functional group compatibility [7] , [8] , [9] , thus limiting applications to the labelling of chemically less elaborate structures. A significant step forward was the development of transition metal-catalysed carboxylations, which substantially reduced previous functional group limitations and thereby increased the scope of these transformations [10] , [11] . A major challenge in isotope labelling, particularly for carbon-14 insertion, is the need for efficient chemistry in the presence of only stoichiometric amounts of labelled CO 2 . An example of a successful dynamic carbon isotope exchange was reported by Audisio and coworkers [12] for the decarboxylation–carboxylation of caesium benzoates catalysed by Cu (Fig. 1b ). Although elegant and direct, full carbon isotope incorporation is challenging because of the equilibrium between labelled and unlabelled CO 2 under the reaction conditions. We and others have also demonstrated the usefulness of isotopically labelled carbon monoxide as a reagent in only stoichiometric or even substoichiometric quantities to access isotopologues of aryl carboxylic acids and esters [13] , [14] , [15] . Nevertheless, as Ba 14 CO 3 represents the primary source of the carbon-14 isotope, an additional CO 2 -to-CO reduction step is required to generate the corresponding labelled carbon monoxide. Fig. 1: Radioactive labelling of aryl carboxylic acids. a Comparison of using CO 2 , CO or MCN as carbon-14 sources for the radiolabelling of aryl carboxylic acids. b Top Modern dynamic CIE method limited to low-carbon isotope incorporations [12] . Bottom Modern strategy for radioactive CRC, limited to only one example and requiring high CO 2 loadings [29] . c Challenges in catalytic reductive carboxylation reactions (CRC). d Proposed method for the late-stage palladium-catalysed electrocarboxylation of aryl electrophiles (this work). Full size image The catalytic reductive carboxylation (CRC) reaction between organometallic species and aryl electrophiles constitutes an alternative route for directly installing a carboxylic group on an aromatic core. These efficient processes, which rely on transition metal-based catalysts including palladium [16] , [17] , [18] , [19] , cobalt [20] , copper [21] , and nickel [22] , [23] , [24] , [25] , [26] , [27] , [28] , nevertheless require a sacrificial reductant to generate a low-valent metal–aryl intermediate and form a new carbon–carbon bond through a CO 2 insertion step. Representative examples of such electron-donating reagents include stoichiometric metal and organic reductants (Mn, Zn, Organic Electron Donors (OEDs), etc. ), or tertiary amines for reductive carboxylations applying visible light photoredox catalysis [16] , [19] , [26] , [27] , [28] . For example, Martin and coworkers reported the use of stoichiometric diethyl zinc with a palladium catalyst for the effective carboxylation of aryl bromides, where high CO 2 pressures were required (up to 10 atm) to avoid the formation of the Negishi side-product [16] . 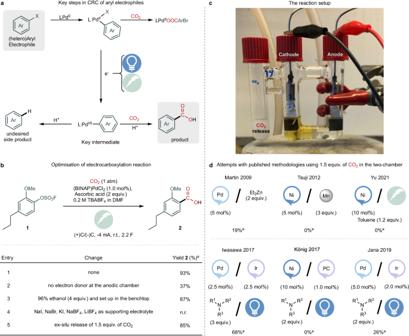Fig. 2: Development of a palladium-catalysed electrocarboxylation method. aKey steps involved in the CRC of aryl electrophiles.bSelected optimisation results. Unless otherwise noted, all reactions were performed in an H-cell with 0.4 mmol of aryl electrophile (1 equiv.) and 3 mL of DMF in each chamber (see SI Section2).cThe reaction setup.dPerforming published CRC methods with 1.5 equivalents of CO2in the two-chamber (see SI Section3)16,17,19,23,25,27.aYields were obtained by1H NMR spectroscopy of a crude reaction mixture with an internal standard. Later, the use of photoredox catalysis in combination with palladium for CRC was disclosed by Martin, Iwasawa, and Jana [17] , [18] , [19] . To prevent parasitic hydrodehalogenation, several additives and 1 atmosphere of CO 2 were required [17] , [18] , [19] . Advances in the use of nickel catalysts for CRC were also successful, first with Tsuji reporting the use of metallic manganese as the reductant, followed by König demonstrating a photoredox setup [25] , [27] . Later, Martin and coworkers adopted Tsuji’s CRC protocol for the radioactive labelling of a single aryl carboxylic acid, although with an excess of 14 CO 2 (Fig. 1c ) [29] . Altogether, it is uncertain whether these contemporary CRC reactions, when run with only (sub)stoichiometric amounts of labelled carbon dioxide, would prove sufficiently effective for accessing the desired labelled aryl carboxylic acids, rather than following alternative but unproductive pathways. Reduction of the metal–aryl intermediate in an electrochemical setup represents an alternative scenario for the generation of the key low-valent species necessary for the carbon dioxide insertion step, with the advantage of avoiding the requirement of stoichiometric reactive reductants. In the early 1990s, Fauvarque, Jutand, and Torii reported the first successful electrochemical CRC using palladium- and nickel-based catalysts. Although seminal, the scope included primarily structurally non-elaborate aryl electrophiles, relying on atmospheric CO 2 pressures and high catalyst loadings (e.g., 7–10 mol% of (PPh 3 ) 2 PdCl 2 ) [30] , [31] , [32] , [33] , [34] . More recently, Yu and coworkers. demonstrated electrochemical nickel-catalysed reductive carboxylation, but relying on high catalyst loading and excess CO 2 , significantly limiting this work’s adaptability in radioactive labelling [23] . Herein, we present an innovative electrochemical approach for the late-stage carboxylation of aryl (pseudo)halides using 13 C- and 14 C-labelled carbon dioxide. Through systematic optimisation, we identified that Pd(BINAP)Cl 2 effectively facilitates the electrocarboxylation reaction under stoichiometric CO 2 concentrations, requiring only 1 mol% catalyst loading (Fig. 1d ). This straightforward yet robust method leverages the ex situ release of CO 2 from BaCO 3 , offering adaptability for the generation of both labelled and unlabelled CO 2 . Notably, our approach avoids the stoichiometric use of highly reactive compounds as reductants. Furthermore, we showcased the practicality of this strategy for the late-stage incorporation of carbon isotopes into complex pharmaceutically relevant molecules in a single chemical step. With minimal investment in electrochemical equipment, our method provides a carbon labelling technology that is anticipated to find widespread use in pharmaceutical drug development. Initial considerations Inspired by the pioneering work of Jutand, Fauvarque, and Torii [30] , [31] , [32] , [33] , [34] , [35] , we set out to develop a general cross-electrophile coupling reaction in an electrochemical setup that provides efficient entry to aryl carboxylic acids with full carbon isotope incorporation (Fig. 2 ). The efficacy of this process hinges on two main factors. First, C–C bond formation through CO 2 insertion into the aryl metal bond should be possible at the targeted low CO 2 concentrations. Second, the aryl-metal intermediate formed must withstand the highly reductive potential required to drive the electrochemical process (Fig. 2a ). In contemporary carboxylation methods, the aryl-metal intermediate in the catalytic cycle generated after the initial oxidative addition step can also participate in off-cycle reactions, such as the hydrodehalogenation reaction in the presence of protons or Negishi couplings in the presence of Et 2 Zn [16] , [36] . These parasitic reactions have hampered efforts to adapt (sub)stoichiometric amounts of CO 2 for CRC reactions. It is essential to maintain a low proton concentration to minimise these undesired side reactions and exploit the advantages of electrochemistry in reducing the proposed aryl-Pd(II) intermediate and facilitating CO 2 migratory insertion. Protons can be present due to acidic motifs or from the oxidation of alkyl amines as sacrificial reductants, which, as for the case of the Pd-catalysed photoredox carboxylation of aryl bromides, requires the addition of two to three equivalents of caesium carbonate as a base [17] , [18] , [19] , [36] . Another approach for controlling the proton inventory in the cathodic chamber is to regulate the proton flux between the cathodic and anodic chambers in a compartmentalised electrochemical cell, thereby avoiding the base additive. In addition, within electrochemical-mediated carboxylation reactions, the redox potential of the on-cycle intermediates is of utmost relevance. Using a strong electron-donating phosphine ligand favours the oxidative addition step; however, it makes the reduction potential of the Pd complex more negative. If catalyst reduction occurs at more negative potentials than the substrate, unfavourable substrate reduction can occur, highlighting the importance of the ligand used. Fig. 2: Development of a palladium-catalysed electrocarboxylation method. a Key steps involved in the CRC of aryl electrophiles. b Selected optimisation results. Unless otherwise noted, all reactions were performed in an H-cell with 0.4 mmol of aryl electrophile (1 equiv.) and 3 mL of DMF in each chamber (see SI Section 2 ). c The reaction setup. d Performing published CRC methods with 1.5 equivalents of CO 2 in the two-chamber (see SI Section 3 ) [16] , [17] , [19] , [23] , [25] , [27] . a Yields were obtained by 1 H NMR spectroscopy of a crude reaction mixture with an internal standard. Full size image Electrocarboxylation optimisation With these considerations in mind, we optimised the Pd-catalysed electrocarboxylation of aryl electrophiles (Fig. 2b ). Our efforts were directed to include the carboxylations of aryl bromides, because of their commercial accessibility, and phenol derivatives, because of the high natural abundance of such substrates. Aryl fluorosulfates were chosen as the pseudo-halide electrophilic partner because of their stability and ease of access from the corresponding phenols. Initial optimisation studies were conducted using the sterically hindered and electron-rich aryl fluorosulfonate 1 (see Supplementary Information Section 2 ). To our delight, the previously depicted limitations could be overcome by exploiting the commercially available catalyst (BINAP)PdCl 2 using an electrochemical approach (Fig. 2b ). Optimum conditions were achieved using an H-cell with tetrabutylammonium tetrafluoroborate (TBABF 4 ) as the supporting electrolyte, carbon paper electrodes (2 cm 2 ), and DMF as the solvent. These conditions resulted in high selectivity and efficiency with only 1 mol% catalyst loading (Fig. 2b , for more detailed optimisation, see SI Section 2 ). The possibility of using a homemade galvanostat (ElectroWare) to apply a constant current of −4 mA further simplified the reaction setup [14] . After optimisation, carboxylic acid 2 was obtained in an 85% yield with only 1.5 equivalents of carbon dioxide, which was released in a three-chamber electro-glassware (Fig. 2c ) using camphorsulfonic acid and barium carbonate (Fig. 2b , entry 5 and see SI Section 2 ). This was achieved without the use of metallic reductants and with the lowest reported catalyst loading for a palladium CRC reaction. Furthermore, only a 8% yield difference was detected when the CO 2 concentration was lowered from 1 atm to 1.5 equivalents (Fig. 2b , entries 1 and 5). The choice of barium carbonate as the CO 2 source provides convenient access to 12 C-, 13 C- and 14 C carbon dioxide. Using an additive, including ascorbic acid, ethanol, or triethylamine, in the anodic chamber was essential for obtaining good yields of the carboxylic acid (see SI Section 2 ). In the presence of the additive, the potential at the cathode is not limited by the rate of the oxidation reaction since such additives should display a lower oxidation potential compared to the solvent, thus obtaining the product with higher yields. To compare our results with previously reported methods, we performed a CRC of 1 with only 1.5 equivalents of CO 2 released in the two-chamber reactor, COware® [16] , [17] , [19] , [23] , [25] , [27] . The respective nickel-catalysed methodologies failed to provide the product with near-stoichiometric CO 2 (Fig. 2d and see SI Section 3 ) [23] , [27] . However, product formation was observed in the reported Pd-catalysed CRC reactions with substantially lower yields while employing higher catalyst loadings [16] , [17] , [19] . Substrate scope Having obtained suitable reaction conditions, we investigated the substrate scope for the Pd-catalysed electrocarboxylation reaction using aryl fluorosulfates and aryl bromides as electrophiles under atmospheric CO 2 pressures (Fig. 3 , cmpds 3 – 10 ). Electron-rich or hindered aryl bromide electrophiles give lower yields due to more demanding oxidative addition, whereas electron-rich or hindered aryl fluorosulfates provide the desired product in good yields. In the case of electron-poor electrophiles, aryl bromides react promptly, whereas aryl fluorosulfates give lower yields, which depend on the reduction potential of the substrate. An electron-withdrawing motif decreases the reduction potential of aryl fluorosulfate, which can lead to substrate reduction as a side reaction. The side-product of this reduction is the corresponding phenol, following a reduction mechanism likely to be similar to that proposed by Jutand et al. for aryl triflates [31] , [34] . The optimised conditions also tolerated a variety of functional groups, including chloride and tosylate substituents, as for compounds 14 and 15 , demonstrating the high chemoselectivity of the reaction. Carboxylation at two positions under slightly modified conditions (–1 mA instead of –4 mA) was feasible, leading to bisphenol-A derivative 18 in 95% yield. Fig. 3: Scope of aryl electrophiles. All reactions were performed using 0.4 mmol of aryl electrophile. All reported yields are an average of at least two runs. RCY is used as an acronym for radiochemical yield. a Reaction performed with 1 atm of 12 CO 2 . b Reaction performed with −2 mA of constant current. c Reaction performed with −1 mA of constant current. d Reaction performed with 5 mol% of pre-catalyst. e Reaction performed with a constant potential. f Reaction performed using ascorbic acid as an additive. g Reaction performed using ethanol as an additive. h Reaction performed once with ascorbic acid as an additive and once using ethanol as an additive. i Reaction performed with the ex situ release of 1.5 equiv. of CO 2 . Full size image With good yields for the reaction using 1 atm of CO 2, we proceeded with the scope using 1.5 equivalents of 13 CO 2 for stable isotopic labelling. Heterocycles are often used as a tool by medicinal chemists to optimise the vital characteristics of a drug candidate, such as solubility, lipophilicity, and hydrogen bonding capacity [37] . 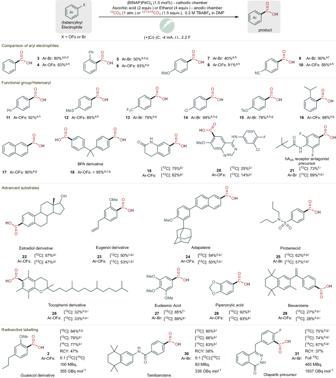Fig. 3: Scope of aryl electrophiles. All reactions were performed using 0.4 mmol of aryl electrophile. All reported yields are an average of at least two runs. RCY is used as an acronym for radiochemical yield.aReaction performed with 1 atm of12CO2.bReaction performed with −2 mA of constant current.cReaction performed with −1 mA of constant current.dReaction performed with 5 mol% of pre-catalyst.eReaction performed with a constant potential.fReaction performed using ascorbic acid as an additive.gReaction performed using ethanol as an additive.hReaction performed once with ascorbic acid as an additive and once using ethanol as an additive.iReaction performed with the ex situ release of 1.5 equiv. of CO2. The reported method provided labelled and unlabelled heteroaryl carboxylic acids in good yields (Fig 3 . cmpds 19 – 21 ). Phenols are often found in nature, some of which have important biological activity; thus, we devised a late-stage derivatization of these natural compounds via the reaction of the phenol with sulphuryl fluoride, which leads to the corresponding aryl fluorosulfonate that can be applied in the electrocarboxylation reaction. With these, a library of natural compounds (derivatives) could be obtained (cmpds 2, 22, 23, 26 – 28 ). Furthermore, the late-stage stable labelling of adapalene ( 24 ), an acne treatment pharmaceutical, and the antineoplastic drug bexarotene ( 29 ) was performed in 50% and 28% yields, respectively. Dynamic carbon isotopic exchange represents a rapid tool to access isotopically labelled active pharmaceutical ingredients (APIs). Nevertheless, this labelling technique generally does not provide full isotopic incorporation because of the dilution of the carbon-labelled CO 2 equilibrium with the released 12 CO 2 [12] , [38] , [39] . With the aim of developing a strategy for the full carbon isotope exchange of carboxylic acids, we envisioned that treating aryl carboxylic acids with the Cu-catalysed decarboxylative bromination developed by Macmillan and co-workers would provide an aryl bromide that can be further transformed to the labelled aryl carboxylic acid by applying the electrocatalytic reaction conditions [40] . Accordingly, the two-step procedure was demonstrated for the late-stage labelling of probenecid, providing the desired compound 25 in 57% yield for the carboxylation step (see Supplementary Information Section 5.2 ). Radioactive labelling is essential for bioactive molecule development and regulatory approval, but its costs can be extensive. To minimise this, the developed method relies on the controlled ex situ release of only 1.5 equivalents of 14 CO 2 and can be easily set up on the benchtop. Moreover, the direct application of Ba 14 CO 3 , the primary carbon-14 reactant, in a late-stage carboxylation reaction avoids additional radioactive steps. The possibility of labelling a compound with carbon-14 was demonstrated in good yields (cmpd 2 ). Next, the late-stage synthesis of a radiolabelled retinoic acid receptor alpha (RARα) agonist, tamibarotene ( 30 ), was demonstrated in 63% yield with only one step of manipulating the radioactive material. Finally, the synthesis of the olaparib precursor 31 was achieved in a satisfactory 67% yield. For the successful application of radiolabelled compounds in the drug development process, distinct molar activities ( A m ) can be required. The use of low A m compounds (230 GBq mol −1 ) can be limited to accelerator mass spectrometry (AMS), but with increased A m other important studies, such as animal mass balance, can be carried out [38] . 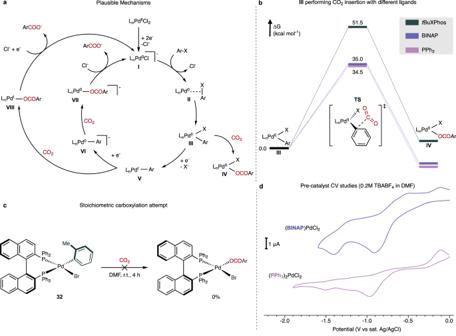Fig. 4: Mechanistic study. aPlausible catalytic cycles (based on reported studies16,36,41, and experimental and computational analyses performed here).bDFT study for carboxylation ofIIIwith different ligands.cReaction of Pd(II) complex32with CO2.dCyclic voltammetry of two different palladium pre-catalysts. 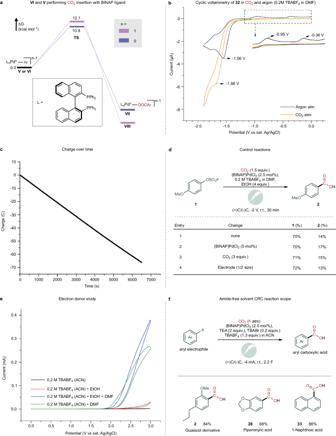Fig. 5: Mechanistic study. aDFT study of the carboxylation ofVandVIwith the BINAP ligand.bCyclic voltammetry of oxidative addition complex32in argon and CO2atmosphere.cConsumed charge during the reaction.dControl reactions.eEffect of adding ethanol in the cyclic voltammetry in DMF and acetonitrile (ACN).fScope of the carboxylation reaction with amide-free solvent. With the described method it is possible to dilute the Ba 14 CO 3 with Ba 12 CO 3 to tune the carbon-14 incorporation, and thus obtain the desired A m , such as for compounds 2 and 30 . In addition, if only Ba 14 CO 3 is used for the gas release, full carbon-14 incorporation is obtained leading to a high- A m compound as demonstrated for compound 31 . Electrocarboxylation mechanistic study After demonstrating the tolerability of the reaction conditions with a wide variety of motifs and applicability to the direct synthesis of carbon-labelled bioactive molecules, efforts were focused on elucidating the reaction mechanism. The reported catalytic cycle consists of an oxidative addition of L n Pd(0) I to the aryl electrophile, leading to the formation of Pd(II) complex III (Fig. 4a ) [16] , [36] , [41] . This complex has been proposed to follow three different routes. Martin and coworkers proposed that the organometallic complex III can perform CO 2 migratory insertion [16] , while Iwasawa coworkers reported that the reduction of III to V occurs prior to the CO 2 insertion [36] . Amatore and Jutand described that the triphenylphosphine ligated III undergoes an overall two-electron reduction to VI before the carboxylation step, which is suggested to occur outside the palladium coordination sphere [41] . We employed density functional theory (DFT) at the B3LYP-D3[IEFPCM] level to compute the barriers for CO 2 α-migratory insertion into complex III with different ligands (Fig. 4b ). With 2-di-tert-butylphosphino−2′,4′,6′-triisopropylbiphenyl (tBuXPhos), PPh 3 and BINAP, the computed energy barriers range from 34 to 51 kcal/mol, which are incompatible with a room temperature reaction. Fig. 4: Mechanistic study. a Plausible catalytic cycles (based on reported studies [16] , [36] , [41] , and experimental and computational analyses performed here). b DFT study for carboxylation of III with different ligands. c Reaction of Pd(II) complex 32 with CO 2 . d Cyclic voltammetry of two different palladium pre-catalysts. Full size image To further validate these results experimentally, we attempted the reaction of aryl-Pd(II) complex 32 with CO 2 at room temperature in DMF (Fig. 4c ). After 4 h, no carboxylation product was observed, confirming that the CO 2 migratory insertion in complex III cannot occur under these reaction conditions. The combined results indicate that the active carboxylation species is not a Pd(II) complex. The palladium’s ability to access odd oxidation states, thus allowing the existence of Pd(I)-species V , depends on the nature of the ligand. DuBois and coworkers demonstrated that bidentate ligands with larger bite angles can stabilise the Pd(I) complex [42] . This is based on electrochemical studies that revealed that [Pd(dppm) 2 ](BF 4 ) 2 undergoes an overall two-electron reduction, whereas 1,2-bis((diphenylphosphino)methyl)benzene (dppx) or 1,2-bis(diphenylphosphino)ethane (dppe) can undergo one-electron reduction [42] . A cyclic voltammetry (CV) study with the (BINAP)PdCl 2 pre-catalyst revealed that the two one-electron reduction peaks are present at −0.85 and −1.35 V vs Ag/AgCl (Fig. 4d and see SI Section 4.2 ), which was also observed by Amatore and Jutand for dppe [41] . In contrast, (PPh 3 ) 2 PdCl 2 , the pre-catalyst employed by Amatore and Jutand for the same transformation, displays one peak corresponding to a two-electron reduction process (Fig. 4d ). In addition to the possibility of accessing a Pd(I) complex, higher stability of the catalyst due to the chelate effect is expected with BINAP. This should inhibit catalyst deactivation due to palladium(0) cluster formation at the operating negative potentials. Next, we computed the barriers for the carboxylation of aryl-Pd complexes V and VI , which showed that both have lower activation barriers than species III , consistent with a CO 2 migratory insertion step at room temperature (Fig. 5a ). To confirm that a low-valent palladium complex is involved in the CO 2 migratory insertion step, we conducted CV studies using the aryl-Pd(II) complex 32 . Interestingly, in the presence of CO 2 , a peak shift was observed at the reduction potential of the Pd(I)/Pd(0) wave (−1.56 V in argon to −1.68 V in CO 2 ) (Fig. 5b ). Furthermore, two oxidation peaks (−0.95 V and −0.36 V) relative to complex 32 in argon are not present in CO 2 atmosphere (Fig. 5b ). These results suggest an interaction between the low-valent palladium complex and CO 2 . To determine if these observations with well-defined species can be translated to the catalytic reaction, we analysed the charge within the course of the reaction for p -methoxy aryl fluorosulfonate using constant potential electrolysis (CPE) (Fig. 5c ). Such an analysis can provide insights into the kinetic profile of an electrochemical reaction, as under a CPE regime, the consumed charge is correlated with the reduction of an analyte, which for the described reaction is complex III . Although the concentration of III decreases with time, a linear decrease is observed, demonstrating that the reaction is of the order of 0 for the palladium catalyst and CO 2 (Fig. 5c and see SI Section 4.5 ). Consistent with this result is the additional observation that the reaction yield and conversion remain constant with double catalyst loading within the same reaction time with a − 2 V (vs. Ag/AgCl) applied potential, indicating that the pre-catalyst concentration does not affect the reaction rate (Fig. 5d ). The same trend was observed for increased CO 2 concentrations, implying that although carboxylation occurs within the palladium coordination sphere, it is not rate-determining. Fig. 5: Mechanistic study. a DFT study of the carboxylation of V and VI with the BINAP ligand. b Cyclic voltammetry of oxidative addition complex 32 in argon and CO 2 atmosphere. c Consumed charge during the reaction. d Control reactions. e Effect of adding ethanol in the cyclic voltammetry in DMF and acetonitrile (ACN). f Scope of the carboxylation reaction with amide-free solvent. Full size image Anodic reaction investigation With a more complete understanding of the carboxylation (cathodic) reaction, we turned our attention to the anodic compartment to elucidate the role of ethanol as an additive. Because of the wider redox window of acetonitrile, it was selected as the solvent of choice for a comparative CV study on the oxidation of DMF and ethanol (Fig. 5e ). This indicates that DMF oxidation is more favourable than ethanol, which leads to the conclusion that the oxidation of DMF is feasible under our reaction conditions in a manner similar to that proposed by Ross et al. to generate a carbonium ion species [43] . Although this oxidation is feasible, trapping the carbonium ion species with a nucleophile leads to an N -alkoxymethyl- N -methylformamide product, which may explain the positive effect of added ethanol on the carboxylation reaction [44] . Thus, the requirement of DMF as a solvent was elucidated: it is the sacrificial reductant. This, in turn, makes the catalytic system a suitable candidate for the use of a non-amide-based solvent. This change is highly desirable and has only been previously reported by Hazari and co-workers using a nickel catalyst. Although sophisticated, it relies on DMAP-OED as an organic reductant, which is sensitive and expensive [26] . Thus, we decided to investigate whether the change of DMF to acetonitrile was feasible. While DMF oxidation occurs under the reported reaction conditions, with acetonitrile, the oxidation is not productive because of the high oxidation potential of the solvent. The use of ascorbic acid as an electron donor was also problematic due to poor solubility. We then envisioned that triethylamine could act as an electron donor, similarly as commonly employed in photoredox catalysis [45] , [46] , [47] . After a small optimisation, it was observed that bromide ions are required for solvent exchange to be viable. This was easily solved by adding TBABr (0.2 equivalents) to the commonly employed TBABF 4 (Fig. 5f ). Thus, under slightly modified conditions, the reaction tolerated the change to a non-amide solvent and allowed the access of aryl carboxylic acids in good yields. Although the use of amide-based solvents for the small-scale synthesis of labelled bioactive compounds does not present an issue, the exchange for a safer solvent and the use of a commercial catalyst in a simple setup lay the foundation for the implementation of catalytic reductive carboxylations in the pharmaceutical industry [48] . In summary, the development of an efficient Pd-catalysed electrocarboxylation method for the late-stage carbon isotope labelling of aryl carboxylic acids is described. This general method can tolerate the use of only 1.5 equivalents of 14 CO 2 , making full radioactive labelling of carboxylic acids attainable in only one radioactive step. In the process, the reaction mechanism was studied, and a key low-valent aryl-Pd complex was proposed to undergo CO 2 migratory insertion in the cathodic chamber, while the DMF participated as the electron donor in the anodic chamber. With a clear understanding of both cathodic and anodic reactions, the use of acetonitrile as an amide-free solvent was feasible. Altogether, we anticipate that our general and mild late-stage carbon label incorporation method will expedite the use of CO 2 as a C 1 synthon for labelling strategies. Moreover, we expect that using a safer solvent with a commercial catalyst in a simple electrochemical setup will promote the implementation of CRC in the pharmaceutical industry.